Metal organic framework-mediated synthesis of highly active and stable Fischer-Tropsch catalysts Depletion of crude oil resources and environmental concerns have driven a worldwide research on alternative processes for the production of commodity chemicals. Fischer–Tropsch synthesis is a process for flexible production of key chemicals from synthesis gas originating from non-petroleum-based sources. Although the use of iron-based catalysts would be preferred over the widely used cobalt, manufacturing methods that prevent their fast deactivation because of sintering, carbon deposition and phase changes have proven challenging. Here we present a strategy to produce highly dispersed iron carbides embedded in a matrix of porous carbon. Very high iron loadings (>40 wt %) are achieved while maintaining an optimal dispersion of the active iron carbide phase when a metal organic framework is used as catalyst precursor. The unique iron spatial confinement and the absence of large iron particles in the obtained solids minimize catalyst deactivation, resulting in high active and stable operation. The growing concerns about oil depletion have spurred worldwide interest in finding alternative feedstocks for important petrochemical commodities and fuels. Fischer–Tropsch synthesis (FTS) is a heterogeneous catalysed polymerization reaction where syngas (a mixture of CO and H 2 ), derived from natural gas, coal or biomass, is converted into a wide spectrum of hydrocarbon chains [1] , [2] , [3] . Cobalt, ruthenium, iron and nickel are all active in FTS, but only iron and cobalt are used industrially. Owing to their high intrinsic activity towards long-chain hydrocarbons, cobalt-based FTS catalysts, remain the preferred catalyst choice for the gas to liquids process. However, Fe-based catalysts have some superior properties over Co-based catalysts, especially for syngas derived from coal or biomass, namely: (i) cheap and widely available compared with Co; (ii) active in the water-gas-shift reaction under typical FTS conditions, enabling the in-situ re-adjustment of the H 2 /CO molar ratio for the conversion of hydrogen lean syngas originating from coal or biomass [1] and (iii) under high-temperature FTS, the product slate of Fe-based catalysts is more directed to short-chain (unsaturated) hydrocarbons and short-chain oxygenates, both among the most important chemical building blocks. The main challenge in the design of Fe-based FTS catalysts lies in overcoming the high deactivation rates because of sintering, carbon deposition and iron phase changes (interconversion of Hägg carbide phase into iron oxides and/or inactive carbides during activation and/or FTS operation) [1] , [2] , [4] , [5] . Under FTS conditions, bulk Fe catalysts display a poor mechanical stability and tend to fragment due to carbon deposits or to density differences between iron oxide and iron carbide phases [6] , [7] . Catalyst fragmentation results in the formation of fines, which lead to reactor operational problems such as pressure drop and/or fouling. A strategy to minimize the nucleation of carbon deposits is to reduce the size of the α-Fe 2 O 3 crystallite precursors. SiO 2 , ZnO, TiO 2 and γ-Al 2 O 3 are often added as structural promoters in order to increase the dispersion of Fe and/or act as spacers. The main drawback of these supports is the formation of mixed oxides that are hardly reducible and therefore non-active for FTS (that is iron silicates, titanates and so on) [8] , [9] , [10] . Carbon supports in the form of activated carbon, carbon nano-fibres (CNF), carbon nano-tubes (CNT), carbon spheres and glassy carbon have been proposed as supports for Fe-based FTS catalysts [2] , [11] . The main advantage of these materials is their chemical inertness, high specific surface area, tunable pore structure and surface chemistry. Generally, carbon-supported catalysts are prepared in a multistep process: (i) carbonization of an organic precursor, (ii) physical or chemical activation of the carbon product, (iii) deposition of the active component by incipient wetness impregnation (IWI) [11] , [12] , ion-exchange [13] or chemical vapour deposition [14] and (iv) thermal treatment involving calcination and/or reduction to form metal nanoparticles. This process is usually non-continuous and the distribution of the active phase is frequently compromised during the high temperature steps, especially when high loadings are targeted. The alternative, direct carbonization of Fe dispersed in different polymers usually results in the formation of iron nanoparticles with a very broad particle size distribution [15] , [16] , [17] . Recently, metal organic frameworks (MOFs) have emerged as promising precursors for the synthesis of nano-materials, because of their unique structure, atomic metal dispersion and textural properties [18] , [19] , [20] , [21] , [22] , [23] , [24] , [25] . For example, by using MOF-5 as a template and furfuryl alcohol (FA) as an additional carbon source, porous carbons have been synthesized as electrode materials for supercapacitors [20] , [25] , whereas Fe 2 O 3 /TiO 2 nano-composites were synthesized from MIL-101(Fe) for photocatalytic water splitting [19] . Herein we report a simple, tunable and scalable MOF-mediated synthesis (MOFMS) strategy for the preparation of exceptionally dispersed Fe nano-particles in a porous carbon matrix. The resulting solids display outstanding FTS performance, with high activity and stability. Synthesis and characterization The Fe-based MOF Basolite F300 was used as a template for the preparation of the different catalysts. Basolite F300 (Fe(BTC), C 9 H 3 FeO 6 ; BTC=1,3,5-benzenetricarboxylate) consists of oxo-centred trimers of Fe 3+ cations connected by trimesate anions [26] . The catalyst containing the highest amount of Fe was prepared by direct pyrolysis of Basolite F300. To tune the Fe to C ratio, FA was used as additional carbon precursor for the synthesis of comparative catalyst samples ( Fig. 1a ). In the latter case, Basolite F300 was first impregnated with a certain amount of FA dissolved in methanol by using IWI. Subsequently, FA was polymerized at 353 and 423 K, for 14 and 6 h, respectively, under N 2 atmosphere. The carbonization of all samples was carried out at 773 K for 8 h under N 2 atmosphere. After this treatment, the materials were passivated at room temperature (RT), using a 2.5% (v/v) O 2 in N 2 for 2 h. The final Fe loading was adjusted by changing the amount of FA used during the IWI step. The synthesized catalysts are denoted as ‘Z-Fe@C’, with Z representing the amount of Fe (wt%) in the catalyst. 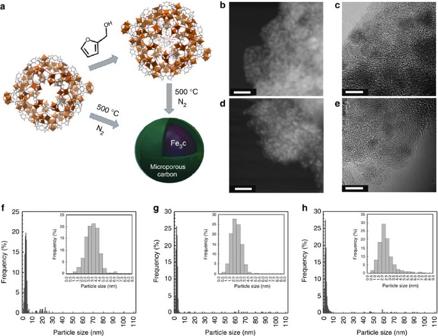Figure 1: MOF-mediated synthesis (MOFMS) strategy and electron microscopy characterization. (a) MOFMS strategy for the Fe-based FTS catalysts: direct pyrolysis of Basolite F-300 and impregnation of the MOF precursor with a carbon source (FA) followed by pyrolysis. (b) High-angle annular dark-field scanning electron (HAADF STEM) micrograph of 38-Fe@C (scale bar, 20 nm). (c) High-resolution (HRTEM) micrograph of 38-Fe@C (scale bar, 5 nm). (d) HAADF STEM of 25-Fe@C (scale bar, 20 nm). (e) HRTEM of 25-Fe@C (scale bar, 5 nm). (f) Particle size histograms obtained from TEM analysis using at least 900 nanoparticles for 38-Fe@C. (g) Particle size histograms obtained from TEM analysis using at least 900 nanoparticles for 31-Fe@C. (h) Particle size histograms obtained from TEM analysis using at least 900 nanoparticles for (iii) 27 Fe@C. Inserts in the histograms (f,g,h) depict the particle size distribution of nanoparticles smaller than 9 nm (representing in every case more than 95% of the nanoparticles counted in the samples). Figure 1: MOF-mediated synthesis (MOFMS) strategy and electron microscopy characterization. ( a ) MOFMS strategy for the Fe-based FTS catalysts: direct pyrolysis of Basolite F-300 and impregnation of the MOF precursor with a carbon source (FA) followed by pyrolysis. ( b ) High-angle annular dark-field scanning electron (HAADF STEM) micrograph of 38-Fe@C (scale bar, 20 nm). ( c ) High-resolution (HRTEM) micrograph of 38-Fe@C (scale bar, 5 nm). ( d ) HAADF STEM of 25-Fe@C (scale bar, 20 nm). ( e ) HRTEM of 25-Fe@C (scale bar, 5 nm). ( f ) Particle size histograms obtained from TEM analysis using at least 900 nanoparticles for 38-Fe@C. ( g ) Particle size histograms obtained from TEM analysis using at least 900 nanoparticles for 31-Fe@C. ( h ) Particle size histograms obtained from TEM analysis using at least 900 nanoparticles for (iii) 27 Fe@C. Inserts in the histograms ( f , g , h ) depict the particle size distribution of nanoparticles smaller than 9 nm (representing in every case more than 95% of the nanoparticles counted in the samples). Full size image The Fe loading of Fe@C varies between 25 and 38 wt% ( Table 1 and Supplementary Fig. 1 ). The textural properties of these samples were evaluated by N 2 adsorption at 77 K and are summarized in Table 1 and Supplementary Fig. 2 . The pyrolysis of Basolite F-300 produces a mesoporous material with a surface area of 130 m 2 g −1 . Hysteresis (type H3) between adsorption and desorption branches at medium pressure (P/P 0 ≈0.4) indicates the presence of mesoporous cavities with a very wide size distribution. In contrast, samples synthesized with additional carbon source are microporous with BET surface areas ranging from 320 to 350 m 2 g −1 . Table 1 Textural characterization of the synthesized catalysts (Fe@C) and MOF precursor. Full size table Transmission electron microscopy on the synthesized catalysts demonstrates the high degree of dispersion of the Fe nanoparticles confined within the porous carbon matrix, regardless the Fe loading ( Fig. 1 and Supplementary Fig. 3 ). Based on these analyses, the mean particle size varies between 2.5 and 3.6 nm for different catalysts. The observed active phase dispersions (up to 39%) have, to the best of our knowledge, never been reported in literature for such highly loaded catalysts. Moreover, X-ray photoelectron spectroscopy (XPS) shows that, despite the high Fe loading and excellent dispersion, only 6–9 wt% Fe is located at the outer surface of the particles, confirming the encapsulation of the Fe phase within the carbon matrix. In situ Mössbauer spectroscopy was applied during the carbonization process to gain insight into the chemical nature of the Fe species formed upon pyrolysis of the MOF precursor ( Fig. 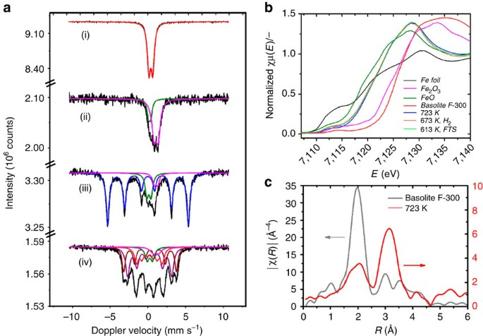Figure 2: Spectroscopic characterization. (a) Mössbauer spectra obtained at 300 K after different successive treatments at 1 bar: (i) Fresh Basolite F-300; (ii) Fe@C obtained after pyrolysis in Ar atmosphere at 723 K (38-Fe@C); (iii) 38-Fe@C after reduction under H2atmosphere at 673 K; and (iv) 38-Fe@C after exposure to syngas (H2/CO=1) at 613 K. (b) X-ray absorption near-edge spectra of iron foil (black); Fe2O3(magenta); FeO (olive); Basolite F-300 at 298 K (red); Fe@C obtained after pyrolysis at 723 K (blue); Fe@C reduced at 673 K by H2/He (10 vol. %, 1 bar; orange); Fe@C after 5 h FTS reaction(613 K, CO/H2= 1, 1 bar; green). (c) EXAFS spectra of Basolite F-300 at 498 K and Fe@C at 723 K. 2a and Table 2 ). The spectrum of the MOF precursor shows the presence of 100% high-spin Fe 3+ in an octahedral environment, in agreement with the literature data [26] . After carbonization, these species are further converted into iron carbide (26% FeC x ) and Wüstite (76% FeO, Table 2 ). Figure 2: Spectroscopic characterization. ( a ) Mössbauer spectra obtained at 300 K after different successive treatments at 1 bar: (i) Fresh Basolite F-300; (ii) Fe@C obtained after pyrolysis in Ar atmosphere at 723 K (38-Fe@C); (iii) 38-Fe@C after reduction under H 2 atmosphere at 673 K; and (iv) 38-Fe@C after exposure to syngas (H 2 /CO=1) at 613 K. ( b ) X-ray absorption near-edge spectra of iron foil (black); Fe 2 O 3 (magenta); FeO (olive); Basolite F-300 at 298 K (red); Fe@C obtained after pyrolysis at 723 K (blue); Fe@C reduced at 673 K by H 2 /He (10 vol. %, 1 bar; orange); Fe@C after 5 h FTS reaction(613 K, CO/H 2 = 1, 1 bar; green). ( c ) EXAFS spectra of Basolite F-300 at 498 K and Fe@C at 723 K. Full size image Table 2 The Mössbauer fitted parameters. Full size table To check the reducibility and the possible formation of more FTS-active carbide species upon exposure to syngas, additional Mössbauer experiments were carried out in situ during FTS ( Fig. 2a and Table 2 ). After exposure of the samples to H 2 at 673 K, most of the Fe atoms (76%) reduce to metallic Fe 0 , with some Fe x C and Fe 2+ structures still present in the spectrum. Exposure of the sample to FTS reaction conditions (H 2 /CO=1) at 613 K for 5 h, converts 86% of the Fe atoms into active Hägg carbide, χ−Fe 5 C 2 , species. We speculate that the remaining Fe x C structures can either originate from the initial carbonization procedure or correspond to very small super-paramagnetic Hägg carbide species. These results demonstrate that the Fe nanoparticles are highly accessible and that almost all metal loaded in the matrix can be utilized for catalysis. The experimental observations from Mössbauer spectroscopy were supported by in situ X-ray absorption spectroscopy (XAS) studies. 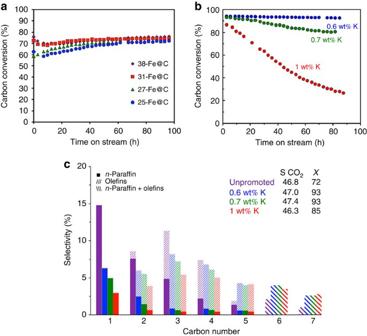Figure 3: Catalytic performance. (a) Time-on-stream evolution of CO conversion for the unpromoted Fe@C catalysts. (b) Time-on-stream evolution of CO conversion for K-promoted 38-Fe@C catalysts. (c) Product distribution after 10 hTOSfor the unpromoted and promoted 38-Fe@C catalysts. Reaction conditions: 613 K, 20 bar, H2/CO=1, and GHSV of 30,000 h−1(space velocity based on catalyst bed volume). Simulating the spectrum of Basolite F-300 yielded parameters listed in Table 3 that closely match the ones deduced from X-ray data refinements for MIL-100(Fe) [26] . The spectrum of Fe@C is markedly different from Basolite F-300. X-ray absorption near-edge spectroscopy analysis on the pyrolysed solid reveals the reduction of Fe 3+ centres of Basolite to Fe 2+ ( Fig. 2b ). Moreover, simulation of the extended X-ray absorption fine structure (EXAFS) results in Fe–O distances close to the ones found in Wüstite ( Table 3 ) [27] . In addition, new scatterers emerge relating to Fe-C at the distance of 2.12 Å, and Fe–Fe at longer distances. Based on the fitting parameters and in line with the Mössbauer data, we conclude that Fe@C consists of a mixture of Wüstite and iron carbides. The reduction of Fe@C catalyst with H 2 ( Table 2 and Supplementary Fig. 4 ) increases the coordination number of Fe–Fe at 2.53 Å, which is consistent with the formation of metallic iron [28] . The exposure of the reduced sample to FTS conditions slightly reduces the contribution of Fe–Fe at around 2.53 Å and at the same time leads to a substantial increase in the long-distance iron scatterers. These results further suggest that Fe 0 formed upon reduction is further transformed to carbidic phase under syngas conditions. However, one should note the difference in H 2 concentrations used in in situ Mössbauer and XAS spectroscopies. The lower concentration in the latter reduces the degree of transformation of Fe@C into Fe 0 . Table 3 Calculated EXAFS refinement parameters. Full size table The electronic properties of Fe in Fe@C were also evaluated by XPS and diffuse reflectance infrared spectroscopy using CO as probe molecule. These experiments were conducted on passivated samples and are summarized in Supplementary Figs 5 and 6 . The surface oxygen functionality of Fe@C was studied from the O1 s core level spectra ( Supplementary Fig. 7 ). Three different types of surface oxygen species can be identified: the band at 530.1–531.1 eV is characteristic of Fe 3 O 4 (refs 29 , 30 , 31 ), whereas the higher energy bands correspond to the presence of surface oxygen groups, namely C=O and COO, respectively [32] . These results suggest that the FA loading significantly increases the relative amount of oxygen groups on the surface of the porous carbon. For example, on 25-Fe@C the relative percentage of oxygenated groups is about 78%, whereas on 31-Fe@C it decreases to 68%. Catalytic results The Fe@C catalysts were tested in the FTS reaction at 613 K, 20 bar, H 2 /CO=1 and gas hourly space velocity (GHSV) of 30,000 h −1 (space velocity based on catalyst bed volume). Owing to the outstanding effect of potassium promotion on iron-based catalyst for FTS, namely improving activity and olefins to paraffins ratio [33] , [34] , [35] , a series of alkali-promoted samples were are also synthesized. The time-on-stream evolution of CO conversion for the un-promoted Fe@C catalysts is presented in Fig. 3a . Independently of the preparation method, all the materials showed very high conversion levels, ranging between 72 and 77% after 90 h on-stream. Under the applied process conditions, the main difference found as a consequence of addition of FA is in the catalyst activation period. Samples containing the highest amount of Fe (38 and 31-Fe@C) display steady-state operation after 30 h on stream, whereas catalysts synthesized with a higher amount of FA show a longer induction period. We attribute these results to slight diffusion limitations as a consequence of their more microporous nature that affect the local H 2 /CO ratio. In spite of these longer activation times, product selectivity after 90 h on stream is similar for all four catalysts ( Supplementary Fig. 8 ). Furthermore, no deactivation was observed. The product spectrum of Fe@C does not deviate from the Anderson–Schulz–Flory distribution, where the chain growth probability changes from 0.40 (for 38-Fe@C) to 0.44 (for 27-Fe@C), depending upon the Fe loading ( Table 4 ). Accordingly, methane selectivity varies from 15.8 to 14.0%, respectively. Selectivity towards olefins (C2–C5) ranges from 14.6 to 15.5% ( Supplementary Table 1 ). Figure 3: Catalytic performance. ( a ) Time-on-stream evolution of CO conversion for the unpromoted Fe@C catalysts. ( b ) Time-on-stream evolution of CO conversion for K-promoted 38-Fe@C catalysts. ( c ) Product distribution after 10 h TOS for the unpromoted and promoted 38-Fe@C catalysts. Reaction conditions: 613 K, 20 bar, H 2 /CO=1, and GHSV of 30,000 h −1 (space velocity based on catalyst bed volume). Full size image Table 4 Catalytic performance of unpromoted Fe-catalysts after 4 h TOS † . Full size table The initial catalytic activities, expressed as iron time yield ( FTY ; mol of CO converted to hydrocarbons per gram of Fe per second), and apparent turnover frequencies ( TOF ) of Fe@C samples are summarized in Table 4 . Furthermore, relevant data from literature for other Fe-catalysts, containing different Fe loadings and supported on carbon nano-fibres [11] (‘X-Fe/CNF’, X: Fe loading) and oxidized carbon nano-tubes [36] (‘20-Fe/O-CNT’), are included in the Table 4 . The catalysts prepared by the MOFMS route display much higher FTY in comparison with X-Fe/CNT. For example, 27-Fe@C is three times more active than 1-Fe/CNF and almost two orders of magnitude more active than 20-Fe/CNF. This remarkable difference is related to the different carbidization degree upon exposure to syngas. Moreover, the encapsulating carbon matrix seems to avoid oxidation of the active carbide phase under reaction conditions [37] . Mössbauer spectroscopy shows that catalysts prepared by the MOFMS approach offer an intimate contact between Fe and C, favouring the formation of χ−Fe 5 C 2 , which is well known to be the most active phase in the FTS process. After 5 h exposure to syngas, about 86% of the Fe atoms in 38-Fe@C are transformed into χ−Fe 5 C 2 , whereas for Fe/CNT this is only 10–20%. FTY of 20-Fe/O-CNT and Fe@C are in the same order of magnitude. Nevertheless, the former shows a very low stability, deactivating by 66% in 50 h (ref. 36 ). Such a poor stability, which is generally observed for systems with larger Fe particles, is often associated with the continuous structural and chemical transformations of the iron phases, as well as to the nucleation of carbon deposits on the catalyst surface [34] . The striking stability of the Fe@C catalysts is attributed to the fact that most Fe nanoparticles are smaller than 9 nm and to the spatial restriction created by the encapsulated carbon. To confirm the stability of Fe@C, additional catalytic tests were performed on 38-Fe@C at higher space velocities (70,000 h −1 ) and lower conversion levels. These results are summarized on Supplementary Fig. 9 and show very stable performance over more than 200 h. The above-mentioned characterization and catalytic performance results highlight the great potential of the MOFMS approach: (i) high iron loadings in FTS catalysts (up to 40 wt%) with (ii) an optimal dispersion of the active phase ( dp Fe <4 nm) that is (iii) formulated in the shape of iron carbides embedded in a porous carbon matrix that prevents unwanted deactivation phenomena. To unravel the effect of pyrolysis conditions on Fe particle size and catalyst activity, we prepared an additional sample starting from the pristine MOF and applying a synthesis temperature of 873 K. The obtained catalyst, with an average Fe particle size of circa 6 nm, showed similar initial TOF of 0.08 s −1 and a longer activation period ( Supplementary Fig. 10 and Supplementary Table 2 ). Furthermore, the catalyst with a bigger Fe particle size, displays a higher chain growth probability and consequently lower selectivity to methane, in agreement with previous studies [11] . Conversion profiles and product distributions of 38-Fe@C catalysts promoted with 0.6, 0.7 and 1.0 wt% of K are shown in Fig. 3b,c , respectively. An Anderson–Schulz–Flory distribution with chain growth probabilities ranging from 0.40 (for the unpromoted catalyst) to 0.7 (for the promoted catalyst with 1 wt% K) is observed ( Supplementary Fig. 11 ). For the unpromoted catalyst the ethene to ethane ratio is about 0.2, whereas for the promoted ones this ratio increases with the amount of K to 1.4, 2.8 and 5.3. Among the promoted samples, an optimal K amount of 0.6 wt% is found: catalysts containing higher amounts of K show a fast deactivation caused by excess of alkali, whereas lower amounts hardly affect the product spectrum. In contrast, 0.6K38-Fe@C displays an optimal selectivity to C2–C5 olefins (20.5% carbon selectivity and 44.6% CO 2 -free selectivity) and an excellent stability with time on stream, next to an increased activity and reduced methane selectivity (5%). We relate the higher activity of the catalyst to an enhancement of the water gas shift functionality and the higher olefin to paraffin ratio to the modulation of the hydrogenation ability, both direct consequences of K promotion. In summary, we have demonstrated that the MOFMS is a promising route for the precise design of Fe-based FTS catalysts. Catalysts prepared following this approach display an intimate contact between Fe and C that facilitates the formation of iron carbides already during the synthesis of the material, which results in very high carbidization degrees. In spite of high Fe loadings that can be realized through this preparation method, the high dispersion of the metal phase and its encapsulation in a highly porous carbon matrix result in an unrivalled activity and exceptional stability. The spatial restriction created by encapsulation seems to minimize sintering and oxidation of the active Hägg carbide phase. The high catalytic activity of the solids here presented is further highlighted when comparing their productivity with that of available data on commercial benchmark catalysts, namely the well-known Ruhrchemie [38] and Sasol [39] catalysts for high-temperature FTS ( Table 5 ). The comparison demonstrates that the MOF-derived solids display productivities, on a total catalyst weight basis, one order of magnitude higher than these benchmarks, even when the MOF-based catalysts contain a lower amount of iron. This simple and potentially universal design strategy opens the door to the controlled manufacture of highly dispersed and stable metal nanoparticles in porous matrices, one of the major challenges in materials science and industrial catalysis [40] . Table 5 Productivities of promoted Fe@C and commercial catalysts. Full size table Synthesis of the Fe@C catalysts The Fe@C catalysts were obtained by carbonization of the MOF precursor. In order to vary the iron loading of the resultant catalyst, a carbon precursor is added to the MOF precursor. In a typical synthesis, a certain amount of FA was dissolved in methanol and impregnated on Basolite F300 by IWI. Subsequently, the FA accommodated inside the pores was polymerized at 353 and 425 K for 14 and 6 h, respectively, under nitrogen atmosphere, using a heating rate of 2 K min −1 . The carbonization was carried out at 773 K for 8 h, under nitrogen atmosphere. The iron loading was tuned by adjusting the amount of FA dissolved in methanol. For the highest loading of iron, Basolite F300 was directly carbonized at 773 K without impregnation with FA. Alkali promotion of the Fe@C catalysts The potassium-promoted catalysts were prepared by IWI. A certain amount of K 2 CO 3 to achieve the desired K promotion level, was dissolved in a mixture of water and methanol (50:50) and impregnated inside the pores of Fe@C. The resultant material was heated up to 353 K for 2 h and carbonized at 773 K for 4 h under nitrogen atmosphere, using a heating rate of 2 K min −1 . Thermogravimetric analysis Thermogravimetric analysis experiments were performed in a Mettler Toledo TGA/SDTA851e apparatus by heating the sample from RT to 1,123 K at a rate of 10 K min −1 in a flow of synthetic air (100 ml min −1 , normal pressure and temperature (NPT)). Nitrogen adsorption measurements Nitrogen adsorption and desorption isotherms were recorded on a QuantaChrome Autosorb-6B at 77 K. Samples were previously evacuated at 373 K for 16 h. The BET method was used to calculate the surface area. Transmission electron microscopy High-angle annular dark-field scanning transmission electron microscopy images were recorded on a JEOL2010F instrument by using an electron probe of 0.5 nm of diameter at a diffraction camera length of 10 cm. High-resolution electron microscopy images were recorded on the same microscope with 0.19 nm spatial resolution. Mössbauer spectroscopy Transmission 57 Fe Mössbauer absorption spectra were collected at 300 K with a conventional constant-acceleration spectrometer using a 57 Co(Rh) source. Velocity calibration was carried out using an α-Fe foil. The Mössbauer spectra were fitted using the Mosswinn 3.0i programme. The spectra were measured at RT, after cooling the sample in the reaction mixture, after each treatment. One Mössbauer spectrum is recorded each time until a satisfactory signal-to-noise ratio is achieved (10–15 h). The dominant Hägg carbide species were evaluated after performing 5 h of FTS reaction at 613 K and 15 bar. The exact time of formation of the Hägg carbide was not investigated. X-ray absorption spectroscopy XAS was performed at BL22, ‘Core level absorption and emission spectroscopies’, beam line of ALBA. The beam line is equipped with Si(111) and Si(311) monochromators and operates in the range of energies between 2.6 and 36 keV. In this particular experiment, the Si(111) monochromator and Rh-coated toroid mirror were employed. The materials were studied using Fe K-edge (ca 7,111 eV) (refs 42 , 43 , 44 ). EXAFS analyses can be found in the Supplementary Figure 4 . Catalytic tests FTS experiments were performed in a 48-flow fixed-bed micro-reactor setup, which allowed running up to 48 reactions in parallel under similar feed composition and process conditions (temperature and pressure). In order to avoid condensation of products at high conversion levels, an inert gas flow (N 2 ) was injected downstream the reactor to each flow. For all experiments, ~10 mg (20 μl) of fresh catalyst with the particle size of 177–420 μm was diluted with 100 μl SiC particles of the same size. Samples were first activated in-situ by pure H 2 at 698 K for 3 h at 3 bar followed by cooling to 613 K under H 2 flow at the same pressure. After increasing the pressure to the process value (20 bar), a 10 cm 3 min −1 flow (NTP) consisting of CO 45 vol. %, H 2 45 vol. % and He 10 vol. % was introduced. A rate of 2 K min −1 was applied for all the heating/cooling steps. A Siemens Maxum Process GC, equipped with multiple columns and detectors in parallel, analysed permanent gases as well as hydrocarbon products up to C7 in the gas phase online. In the first column ( Carboxen 1010, 10 m × 0.32 mm) N 2 , CO, CH 4 and CO 2 were separated at 333 K and analysed by Thermal conductivity detector (TCD). In the second column (Al 2 O 3 /KCl, 10 m × 0.32 mm) with flame ionization detector (FID) detection, separation between all C1–C4 components was achieved at 434 K. CO conversion (%), carbon selectivity (%), molar fraction (-) of each product are defined in Supplementary Table 2 . Catalytic activity is expressed as Fe time yield ( FTY ), defined as the number of CO moles converted to hydrocarbons per gram of Fe per second. How to cite this article : Santos, V. P. et al . Metal organic framework-mediated synthesis of highly stable and active Fischer–Tropsch catalysts. Nat. Commun. 6:6451 doi: 10.1038/ncomms7451 (2015).